Hybrid multiphoton volumetric functional imaging of large-scale bioengineered neuronal networks Planar neural networks and interfaces serve as versatile in vitro models of central nervous system physiology, but adaptations of related methods to three dimensions (3D) have met with limited success. Here, we demonstrate for the first time volumetric functional imaging in a bioengineered neural tissue growing in a transparent hydrogel with cortical cellular and synaptic densities, by introducing complementary new developments in nonlinear microscopy and neural tissue engineering. Our system uses a novel hybrid multiphoton microscope design combining a 3D scanning-line temporal-focusing subsystem and a conventional laser-scanning multiphoton microscope to provide functional and structural volumetric imaging capabilities: dense microscopic 3D sampling at tens of volumes per second of structures with mm-scale dimensions containing a network of over 1,000 developing cells with complex spontaneous activity patterns. These developments open new opportunities for large-scale neuronal interfacing and for applications of 3D engineered networks ranging from basic neuroscience to the screening of neuroactive substances. Spatiotemporal neuronal activity patterns are the fundamental representation of information within the nervous system. The complexity of real neural circuits and experimental challenges associated with in situ pharmacological manipulation and light scattering have motivated the development of simplified and accessible in vitro experimental systems such as neural cell and slice cultures where many aspects of natural neural dynamics are reproduced [1] . Such cultures retain many morphological, pharmacological and electrical properties of in vivo cortical networks [2] and allow much more detailed observation and manipulation options than available for intact brains [3] , [4] , usually through the use of planar multielectrode arrays (MEAs) [5] . These powerful combined abilities to observe and/or manipulate network-wide activity together with access to synaptic physiology, have already led to discoveries on universal characteristics of neural circuits that were later reaffirmed in an in vivo setting (for example, homeostatic rescaling [6] ). Nevertheless, two-dimensional cultures capture only a limited facet of central nervous system connectivity and local microenvironments’ biological and biophysical properties derived from cell-matrix interaction [7] , motivating the recent development of 3D models [8] , [9] , [10] . The development of 3D cultures and the associated interface technology has not yet advanced to a stage where it allows the generation and detailed monitoring of realistic central nervous system-like network models, with major challenges remaining on both fronts. Although early attempts at extending MEA technology to 3D were demonstrated [11] , [12] , it is generally accepted that optophysiology methods are optimally suited for the required non-contact, volumetric interfacing. Indeed, two-photon laser scanning microscopy (TPLSM) neuronal imaging using calcium-sensitive dyes or genetically-encoded indicators [13] is routinely used to image the activity of small neuron ensembles in vivo . However, scanning methods cannot generally achieve dense 3D imaging—with the exception of technically advanced multiplexing schemes [14] , most systems developed for rapid TPLSM imaging were generally based on sparse sampling of space [15] , [16] , [17] (which is movement sensitive), whereas dense volumetric image acquisition at rates of 10 Hz or more, as required for action potential detection [18] , is still generally considered a major challenge. We developed a scanning-line temporal-focusing (SLITE) microscope for rapid volumetric multiphoton fluorescence imaging of a large field of view and here we show dense microscopic imaging of a novel 3D spontaneously active network with brain-approximating characteristics grown in vitro in an extracellular matrix-like hydrogel. In temporal focusing (TF) nonlinear microscopy, the laser pulse’s duration, rather than its spatial dimensions, is manipulated (‘focused’) to generate optically-sectioned illumination of thin planes [19] , [20] , [21] , lines [22] , [23] , [24] or flexible patterns [25] , [26] , [27] inside a 3D volume without the need for tight spatial focusing. Line illumination geometry, also referred to as simultaneous spatial and TF [23] , was demonstrated to be suitable for rapid imaging [22] and to have excellent sectioning capabilities inside a scattering medium [28] . To effectively excite a long line simultaneously, our SLITE microscope uses a regeneratively amplified ultrafast laser source (RegA 9000, Coherent) which provides τ a =200 fs pulses at f a =150 kHz repetition rate and an average power of 600 mW (4 μJ per pulse). Compared with standard Ti:Sapphire lasers, which are commonly used for TPLSM, and provide τ s= 100 fs pulses at f s =80 MHz repetition rate (7.5 nJ per pulse), the amplified laser enhances two-photon absorption by a factor of for identical average power. Moreover, since laser power remains a limiting factor for parallelized multiphoton excitation techniques even when an amplified laser source is used, our setup is based on a new light-efficient design that also introduces the new ability to seamlessly switch between SLITE and TPLSM scanning modes; having this bi-modal imaging capability in the same sample turns out to provide crucial synergistic benefits for practical tissue imaging. Considering the unique constraints and requirements imposed by the dynamic structure of developing bioengineered tissue cultures, SLITE microscopy appears to be a particularly suitable imaging approach for monitoring their activity: unlike other state-of-the-art multiphoton imaging systems [15] , [16] , [17] , our system creates structured, dense 3D stacks rather than rapid serial point-scans that require planning, optimizing and readjusting of sparse cell-crossing complex scan trajectories. Its excellent performance in lightly-scattering bioengineered tissue is limited primarily by the detection camera performance and imaging speed limits—200 frames per second in our experiments, and potentially orders-of-magnitude faster in future implementations. Rapid 3D SLITE-multiphoton microscope design The dual-mode SLITE-multiphoton microscope schematic and method of operation are shown in Fig. 1 . It is based on a new design concept for TF microscopy: whereas previous systems [19] , [20] , [21] , [22] , [23] , [24] , [25] , [26] , [27] used reflective gratings where the light propagation direction is changed after being diffracted, light propagation in this system is along a single linear axis ( Supplementary Note 1 ). This design is based on the use of a custom transmission diffraction grating, mounted between two prisms (dual-prism grating, DPG) and has three fundamental advantages. First, it enables a simple, seamless switch between TF and TPLSM, which were integrated here into a single system for the first time. Switching to SLITE mode simply requires introducing a DPG+cylindrical lens module instead of the scan lens, and rotating a dichroic mirror that deflects the emitted fluorescence signal towards an EMCCD camera ( Fig. 1a ). Second, since the imaging system is limited by pulse energy, the DPG’s enhanced diffraction efficiency (85% in our setup) relative to reflective diffraction gratings (typically 50–70%), provides a major improvement in system characteristics (see also Supplementary Fig. 1 ). Third, DPG-based TF setup enables to remotely scan the focal plane [29] , which may be useful in future applications. Plane imaging is achieved by lateral scanning of the illuminated line by operating one of the microscope’s galvanometric mirrors ( Fig. 1d , xy plane and Supplementary Movie 1 ); axial scanning is achieved by moving the objective lens using a piezoelectric device ( Fig. 1d , yz plane and Supplementary Movie 1 ). When a large field-of-view objective lens is used ( × 10, NA=0.45, Zeiss), the fundamental axial sectioning in our system is 13 μm FWHM ( Fig. 1b , consistent with a recent model [28] ). The dynamic elements of the system—scanning mirror, camera, piezoelectric device and a Pockels cell that attenuates the laser beam intensity, are synchronized to perform dense volumetric imaging ( Supplementary Fig. 2 ). 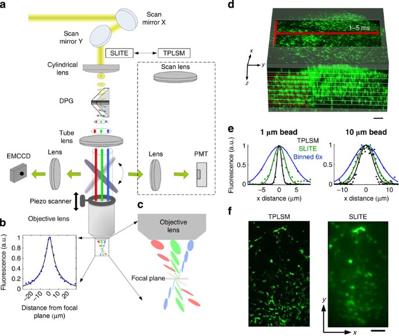Figure 1: Dual-mode TPLSM-SLITE microscope. (a) Optical scheme: in the single-axis SLITE mode a transmission grating diffracts the laser beam, but the central wavelength (800 nm) maintains its propagation direction due to refraction by the prism facets. For TPLSM, a scan lens replaces the cylindrical lens and DPG and the dichroic mirror redirects the fluorescence toward a photomultiplier tube (dashed line). (b) SLITE axial sectioning, measured values (dots) versus predicted28(line). (c) Expanded view of light propagation in focal volume. (d) A 3D imaging geometry: rapid functional SLITE imaging is performed in the volume first acquired using ‘structural’ TPLSM. A temporally focusedxaxis illuminated line is rapidly scanned in theyaxis, while the objective is scanned axially. (e) Measured optical profiles of 1 μm (left) and 10 μm (~cell-sized, right) fluorescent beads, using TPLSM (black dots), SLITE (green dots) and SLITE with 6 × 6 camera pixel binning (blue dots). Solid lines are Gaussian fits. (f) Z-projections of volumes acquired by TPLSM (0.5 Hz acquisition rate) and SLITE (200 Hz acquisition rate). Scale bar, 100 μm. Figure 1: Dual-mode TPLSM-SLITE microscope. ( a ) Optical scheme: in the single-axis SLITE mode a transmission grating diffracts the laser beam, but the central wavelength (800 nm) maintains its propagation direction due to refraction by the prism facets. For TPLSM, a scan lens replaces the cylindrical lens and DPG and the dichroic mirror redirects the fluorescence toward a photomultiplier tube (dashed line). ( b ) SLITE axial sectioning, measured values (dots) versus predicted [28] (line). ( c ) Expanded view of light propagation in focal volume. ( d ) A 3D imaging geometry: rapid functional SLITE imaging is performed in the volume first acquired using ‘structural’ TPLSM. A temporally focused x axis illuminated line is rapidly scanned in the y axis, while the objective is scanned axially. ( e ) Measured optical profiles of 1 μm (left) and 10 μm (~cell-sized, right) fluorescent beads, using TPLSM (black dots), SLITE (green dots) and SLITE with 6 × 6 camera pixel binning (blue dots). Solid lines are Gaussian fits. ( f ) Z-projections of volumes acquired by TPLSM (0.5 Hz acquisition rate) and SLITE (200 Hz acquisition rate). Scale bar, 100 μm. Full size image Tissue-engineered 3D neuronal ‘optonets’ Optimized protocols were developed for generating and maintaining the long-term growth and physiological viability of high-density bioengineered 3D networks of embryonic dissociated rat cortical cells inside an optically-accessible scaffold ( Supplementary Fig. 3 ). Dissociated cell populations containing both neurons and glia encapsulated at high densities of 40,000–60,000 cells μl −1 in Matrigel extracellular matrix-like hydrogel scaffold, were maintained for 5–42 days in a medium containing a custom cocktail of growth supplements and neurotrophic growth factors that supported network development ( Supplementary Movie 2 ). To characterize the networks’ components and their viability, we applied a series of specialized stains which were imaged using a confocal microscope. Using whole-gel differential immunostaining for glia (S100) and neurons (βIII-tubulin), we established that both cell types are growing in the network ( Fig. 2a and Supplementary Movie 3 ), with a stable 1:4 neuron:glia ratio reached by day 21 ( Fig. 2b and Supplementary Fig. 4 ), indicating a fundamental similarity to normal cortical tissue. Both cellular subpopulations demonstrate a very high degree of cellular viability (>95% following network stabilization at day 14, Fig. 2c,d , Supplementary Fig. 5 and Supplementary Movie 4 ), which was found to be critically dependent on glial cell proliferation. Short treatment with the antiproliferative agent arabinofuranosyl cytidine (ARA-C) led to collective network degeneration which began during the second week of culturing ( Fig. 2b,d,f , red lines; Supplementary Fig. 6 ). To study the characteristics of synaptic connectivity, fluorescently labelled synaptic proteins (Cerulean tagged SV2 and EGFP tagged PSD95) were time-lapse imaged over several days ( Fig. 2c and Supplementary Movie 5 ). Neurons in the network develop a multitude of synaptic connections that in mature networks have spine densities (0.5±0.1 μm −1 ; three experiments, DIV16–31, n =7 neurons, 2,972 spines) comparable with these reported in vivo at similar developmental stages (0.3–0.6 μm −1 ) [30] . Younger preparations (DIV14–18) showed extensive growth and synaptogenesis, with a multitude of elongating axons and dendrites that freely invaded the embedding Matrigel, led by motile growth cones, and formed complex networks and new synapses. Older (DIV23–35) cultures exhibited milder yet apparent growth dynamics and more stable synaptic connections. Cell growth and network evolution change the scattering characteristics of the sample, which gradually became more turbid, remaining far less scattering than cortical tissue [31] ( Supplementary Fig. 7 ). Networks generated spatiotemporally complex spontaneous activity patterns ( Supplementary Movie 6 ) as early as DIV 5, whose activity rate and patterns also varied systematically with network age ( Supplementary Fig. 8 ). 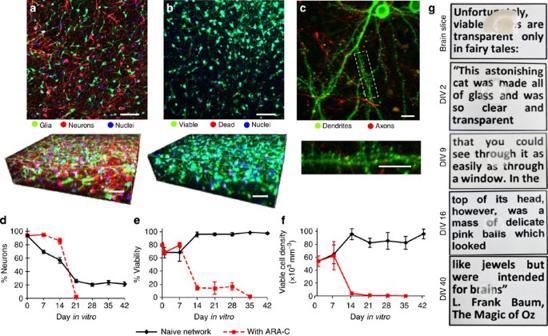Figure 2: Development and characteristics of 3D hydrogel-encapsulated dense neural network. Embryonic rat cortical dissociated cells were encapsulated in a Matrigel scaffold and allowed to create a spontaneous network. Images shown and analysed in (a–f) were taken using a confocal microscope. (a) Cellular content immunostains for neurons (red, βIII tubulin), glia (green, S100) and nuclei (blue, DAPI), showing confocal sections (a,b,c) and 120-μm-thick 3D stacks (a,b). (b) Viable (green, calcein) versus dead (red, ethidium homodimer) cells in the network versus total nuclei (blue, DAPI). (c) Synaptic morphology in neurons virally transfected with the synaptic vesicle protein SV2 (red) and the postsynaptic density protein PSD95 (green). Bottom panels: weeklyin vitrodevelopment characteristics of the neuronal cell content (d), viability (e), and network density (f, number of nuclei of viable cells per mm3) when glial proliferation is normal (black lines) or inhibited using ARA-C (red lines). Broken line indicates disintegrated network, error bars indicate s.e.m. (g) Characteristic scattering by 500-μm-thick rat cortical brain slice and characteristic optonets photographed over text. Scale bars, 50 μm (a,b) or 15 μm (c). Figure 2: Development and characteristics of 3D hydrogel-encapsulated dense neural network. Embryonic rat cortical dissociated cells were encapsulated in a Matrigel scaffold and allowed to create a spontaneous network. Images shown and analysed in ( a – f ) were taken using a confocal microscope. ( a ) Cellular content immunostains for neurons (red, βIII tubulin), glia (green, S100) and nuclei (blue, DAPI), showing confocal sections ( a , b , c ) and 120-μm-thick 3D stacks ( a , b ). ( b ) Viable (green, calcein) versus dead (red, ethidium homodimer) cells in the network versus total nuclei (blue, DAPI). ( c ) Synaptic morphology in neurons virally transfected with the synaptic vesicle protein SV2 (red) and the postsynaptic density protein PSD95 (green). Bottom panels: weekly in vitro development characteristics of the neuronal cell content ( d ), viability ( e ), and network density ( f , number of nuclei of viable cells per mm 3 ) when glial proliferation is normal (black lines) or inhibited using ARA-C (red lines). Broken line indicates disintegrated network, error bars indicate s.e.m. ( g ) Characteristic scattering by 500-μm-thick rat cortical brain slice and characteristic optonets photographed over text. Scale bars, 50 μm ( a , b ) or 15 μm ( c ). Full size image Rapid volumetric functional imaging To volumetrically image spontaneous network physiology, we used the combined structural-functional TPLSM-SLITE approach to image networks that were bath-loaded with the fluorescent calcium indicator Fluo-4-AM ( n =14, DIV6–32). An imaging experiment began by acquiring TPLSM structural images of the tissue (as in Fig. 1d ) followed by the acquisition of 10,000–150,000 3D-image SLITE movies of the same volume. Individual experiments used either a Zeiss × 10 NA=0.45 objective (FOV: 600 × 1000 μm 2 , n =7 networks with 922±176 cells in FOV), or an Olympus × 20 NA=0.5 objective where the xy field of view is roughly halved (FOV: 250 × 500 μm 2 , n =7 networks with 201±83 cells in FOV), while resolution is doubled. As the imaging rate bottleneck was EMCCD acquisition rate, we reduced the spatial resolution to 6 μm per pixel by binning adjacent pixels: binning reduced the SLITE spatial resolution but left cell-sized details roughly unchanged ( Fig. 1e ), while allowing the system to reach rates of 200 frames per second for large field-of-view imaging ( Fig. 1f , and see Methods for details). Imaged volumes had depths of 150–300 μm (limited by dye penetration) and in representative networks contained 327, 1,462 and 966 cells ( Fig. 3 ; first network imaged at high magnification, all three networks were imaged at 200 frames per second and 10 volumes per second). Following cell segmentation, the high temporal resolution SLITE movies were converted to dF/F vectors for the entire network ( Fig. 3d–f , each row describes the activity of a single active cell over time at 10 samples per second), and calcium transients were detected. Approximately 30% cells in these networks showed functional activity (110/327, 384/1,462 and 346/966, respectively for Fig. 3 networks, Supplementary Movie 7 , 29±13% for the 14 networks): activity traces of the entire network ( Fig. 3d–f ) as well as of individual cells ( Fig. 3g–h , inset in Fig. 3h shows an average calcium transient from a single trace, with best-fit exponential template), showed a high degree of spatiotemporal heterogeneity, not limited to the characteristic burst-dominated activity typically seen in two-dimensional networks using MEAs [32] . Spontaneous multi-neuronal synchronized activity events were also occasionally observed ( Fig. 3f,i , six events detected, Supplementary Movie 8 ). Different bursts generally did not engage the same cells and their underlying propagation dynamics may nevertheless reflect an underlying spatiotemporal structure (for example, Fig. 3i , Supplementary Movie 9 ). 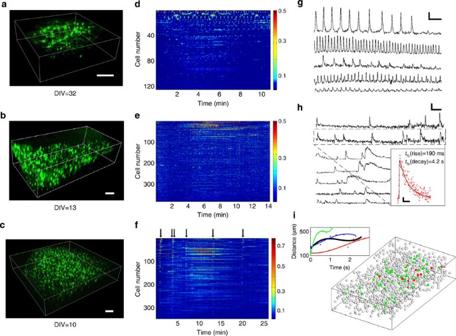Figure 3: Networks’ functional imaging. (a–c), Volumetric structural images of three networks. Imaged volume dimensions were 200 × 500 × 150 μm3(a, 327 cells) and 600 × 1,000 × 200 μm3(bandc, 1,462 and 966 cells, respectively). Scale bar, 100 μm. (d–f) dF/F pseudo-color plots for active cells in each network shown ina–c(121, 384 and 346 cells ind,eandf, respectively). Cells are organized according to their maximal dF/F value. Arrows infmark network activity bursts. (g–h) dF/F traces of several cells from networks shown inaandb, respectively. Scale bars forgandhare 60 s and dF/F=0.25, and 60 s and dF/F=0.5, respectively. Inset inhshows an averaged calcium transient for the marked reference trace (red dots), with best-fit exponential template (solid black line), and rise and decay times to half of the signal maximum (scale bar, 4 s and 0.1 dF/F). (i) Demonstration of a burst spatiotemporal structure in imaged networkcis shown. Each sphere represents a cell; red spheres represent cells that fire in the first 1.5 s of the activity (12/50 cells), green spheres represent all the other active cells. Inset shows the time-dependent average distance of all active cells from the burst origin for four different bursts (dots), with fitted trend lines. Figure 3: Networks’ functional imaging. ( a – c ), Volumetric structural images of three networks. Imaged volume dimensions were 200 × 500 × 150 μm 3 ( a , 327 cells) and 600 × 1,000 × 200 μm 3 ( b and c , 1,462 and 966 cells, respectively). Scale bar, 100 μm. ( d – f ) dF/F pseudo-color plots for active cells in each network shown in a – c (121, 384 and 346 cells in d , e and f , respectively). Cells are organized according to their maximal dF/F value. Arrows in f mark network activity bursts. ( g – h ) dF/F traces of several cells from networks shown in a and b , respectively. Scale bars for g and h are 60 s and dF/F=0.25, and 60 s and dF/F=0.5, respectively. Inset in h shows an averaged calcium transient for the marked reference trace (red dots), with best-fit exponential template (solid black line), and rise and decay times to half of the signal maximum (scale bar, 4 s and 0.1 dF/F). ( i ) Demonstration of a burst spatiotemporal structure in imaged network c is shown. Each sphere represents a cell; red spheres represent cells that fire in the first 1.5 s of the activity (12/50 cells), green spheres represent all the other active cells. Inset shows the time-dependent average distance of all active cells from the burst origin for four different bursts (dots), with fitted trend lines. Full size image The advent of cellular- and molecular-level optophysiology tools in recent years has generated much interest in the development of optically-clear or minimally-scattering preparations and tools for providing simplified optical access to large extended functional networks. However, exciting optical clearing approaches like Clarity [33] , are currently limited to nonvital applications, whereas large-scale light-sheet imaging [34] approaches are limited to lightly-scattering samples where illumination light can be delivered from the side. Our approach provides a functional cellular-resolution interface with large neural populations (containing upwards of 1,000 cells) inside a viable, functional and extended (centimeter-wide) bioengineered neural network. The 3D ECM-like growth environment and conditions were found to support the spontaneous development of morphological and physiological characteristics that are brain-like in terms of cellular and synaptic densities (not shown in earlier in vitro studies), neuron:glia ratio (1:4, similar to human cortex [35] ), dependence of viability on glial proliferation ( Fig. 2 and Supplementary Fig. 6 ) and the emergence of spontaneous electrophysiological activity ( Fig. 3 and Supplementary Fig. 8 ). SLITE microscopy was then shown to allow rapid, cellular-resolution dense imaging (without the need for sparse spatial sampling) inside relatively large mm-scale volumes with tight axial sectioning; the use of an amplified femtosecond laser source enables extended line excitation with a good signal-to-noise ratio. Moreover, the new design combining TPLSM and SLITE provides both high spatial resolution images and high temporal resolution movies of the same volume, benefitting from the disparate strengths of each modality in a single imaging session ( Supplementary Movie 8 and Supplementary Fig. 9 ). Unlike other state-of-the-art multiphoton imaging systems [15] , [16] , [17] , SLITE microscopy does not rely on rapid serial point-scanning (see Supplementary Table 1 for comparison), and thus fundamentally moves the imaging bottleneck from planning and optimizing complex scan trajectories to the performance limits of the detection camera collecting the light emitted from the illuminated focal plane (200 frames per second in our experiments). When combined with contemporary camera systems operating at multi-kHz frame rates it is well poised for tackling the challenges of ultra rapid multiphoton imaging in a large network, which is required for millisecond-accurate imaging using calcium [17] or even voltage [36] indicators. Dense spatial sampling has additional advantages in the context of neural imaging, enabling simpler correction of movement artifacts than hopping systems, and the ability to monitor activity in developing, highly-motile networks. Although presented here in the context of imaging a bioengineered neural tissue, SLITE and related rapid TF methods [21] , [37] can clearly also be used to image neuronal activity in other lightly-scattering preparations such as c-elegans [37] and zebrafish. Technical adaptations could potentially also have an important role in imaging cortical network activity patterns in vivo and may find additional applications in other fields of biomedicine where relatively rapid dense volumetric imaging is advantageous, including moving tissues such as the heart, and super-resolution imaging, where rapid planar acquisition may significantly enhance imaging rate [38] . Further development and refinement of this new type of in vitro neural interfacing technology using, for example, the wide variety of optogenetic probes for monitoring [13] , [39] and/or controlling [40] neuronal activity using complementary photostimulation systems [41] , [42] , could lead to a new generation of optically accessible and sensitive bioengineered networks or ‘optonets’, where even 3D growth and connectivity could potentially be optically guided [43] , [44] . Such an optical-neuronal interface may find applications in the in vitro study of neuronal computations, testing of pharmacological agents and their effects on network activity patterns, and could potentially also lead to a new generation of bio-hybrid medical devices and applications. Optical system design The dual SLITE-TPLSM system was designed for rapid functional imaging of a large field of view with single cell resolution, and is based on the development of a single-optical-axis TF setup, to enable easy combination of a TF microscope with TPLSM or other optical modalities. A regeneratively amplified laser source (RegA 9000, pumped and seeded by a Vitesse duo; Coherent) provides 800 nm, 200 fs pulses with up to 1.5 μJ per pulse (measured at the sample plane) at 150 KHz repetition rate. Illumination power is controlled by a Pockels cell (Conoptics), and a beam expander is used to expand the laser beam cross section. For SLITE microscopy, the beam is scanned in the line lateral direction using a single scanning mirror (Cambridge Technologies), focused by a cylindrical lens ( f =100 mm) on a transmission grating surface, and diffracted by the DPG (Wasatch Photonics). The prism angles (48° × 42° × 90°, BK7 glass) and the diffraction grating groove density (1,200 lines mm −1 ) are designed to refract and diffract the laser’s central wavelength (800 nm) toward the same direction of the incoming light propagation, and have an efficiency of 85% for both polarization states. The microscope’s tube (Nikon) and objective lenses (Zeiss × 10 NA=0.45, Olympus × 20 NA=0.5; actual magnifications=12 and 22, respectively due to the different tube), mounted in a 4f configuration, image the grating surface onto the objective focal plane—where a temporally focused line is obtained. We image this line using an epi-detection scheme ( Fig. 1a ), where the fluorescence light is reflected by a dichroic mirror (Chroma) towards an EMCCD camera (iXon 885, Andor Technology). Each line scan cycle is synchronized with one image acquisition ( Supplementary Fig. 2 ). The camera’s maximal imaging rate is 200 frames s −1 for 100 lines per image reading, and therefore we also used 5 ms for the line scanning. The objective lens was moved axially by a piezoelectric device (Nanomotion) with rates of up to 20 Hz and controlled amplitude of up to several millimetres, with resolution of 50 nm. After picking an axial scanning amplitude and rate, the planar images number per cycle (usually 10–20 images per 100 ms, and axial range of 150–300 μm in our experiments) defines the axial resolution. To minimize the tissue exposure to light, the Pockels cell blocked the laser beam intensity when the piezoelectric device returned the objective lens to its initial position at the end of volumetric scanning cycle ( Supplementary Fig. 2 ); thus only 90% of the images contained information. Switching from SLITE microscopy to TPLSM is simply done by replacing the cylindrical lens and DPG with a scan lens ( Fig. 1a ), two galvanometric mirrors are used to scan the beam, and the dichroic mirror is rotated to direct the fluorescence signal toward a photomultiplier tube (Hamamatsu). TPLSM images were acquired using the ScanImage software [45] , typically with 512 × 512 pixels and a 4 ms per line rate. Therefore, a single planar image acquisition time was 400 times longer than SLITE image. Preparation of 3D neural cultures The animal experiments and procedures were approved by the Institutional Animal Care Committee at Technion—Israel Institute of Technology and were in accord with the National Institutes of Health Guide for the Care and Use of Laboratory Animals. We removed and diced cortical tissue from embryonic day 18 (E18) Sprague Dawley rats in cold phosphate-buffered saline (PBS) solution with 20 mM glucose, mechanically dissociated neural cells (by forcing a few times through a pipette), and filtered the suspension using a 70 μm cell strainer (Biologix). A total of 1.2–1.8 million cells were encapsulated in 30 μl Matrigel scaffold (Growth factor reduced, BD Biosciences). Culturing media was composed of Minimal Essential Media (MEM, Sigma) containing 17 mM glucose, 100 μl ml −1 of NU Serum (BD Biosciences), 30 mg ml −1 of L-glutamine (Sigma), 1:500 B-27 supplement (Gibco), 50 ng ml −1 of nerve growth factor (NGF, Alomone labs), 10 ng ml −1 of brain-derived neurotrophic factor (BDNF, R&D systems), 25 μg ml −1 of insulin (Sigma), and 2 μg ml −1 of gentamicin. Half the volume of the culturing media was replaced twice a week. In a second group of cultures, 3 μM of arabinofuranosyl cytidine (ARA-C, Sigma) to inhibit glial cell proliferation was added once at DIV3. Staining and image analysis For whole-gel viability staining, a MEM solution containing 0.4 μM of ethidium homodimer (Sigma), a nucleic acid fluorescent tag designed to stain dead cells red, 8 μM calcein (Sigma), which stains live cells green and 6 nM of 4′,6 diamidino-2-phenylindole (DAPI, Sigma), a fluorescent tag that stains the nuclei of all cells blue was added. Cultures were incubated for 2.5 h at 37 °C while shaking, and then washed. Imaging was performed using a confocal microscope (Zeiss, LSM 700). Imaris software (Bitplane) was used for counting the total number of cells visible in one plane. The counts of the live and dead cells, and total nuclei in each image were used to calculate the vitality percentage for each sample: each week in vitro n =6–10 naive networks (3–5 cell extractions × 2 replicates each) and n =2–8 ARA-C treated cultures (1–4 cell extractions × 2 replicates each) were evaluated. Viable cell density was evaluated by counting nuclei in confocal image stacks of 320 × 320 × 50 μm ( n =3–8 naive and n =2–8 ARA-C treated networks for each week), and multiplying by the corresponding viability rate. For whole-gel differential immunostaining, cultures were fixated for 2 h using a 4% paraformaldehyde solution in PBS, followed by 4 h of permeabilization and a blocking process in 0.3–1% Triton and 4% fetal bovine serum solution in PBS. The cultures were washed, and the primary antibodies Mouse-Anti Beta III Tubulin (1:400, Promega), a marker of neuronal cells, and Rabbit-Anti S100 (1:200, Sigma), a marker of glial cells, were added, and incubated overnight at 4 °C. Cultures were washed and secondary antibodies, CY 3 Conjugated Goat-Anti-Mouse Immunoglobulin (1:100, Jackson) and Dylight 488 Conjugated Goat-Anti-Rabbit IgG (1:100, Jackson), were added along with DAPI (6 nM, Sigma), designed to stain the nuclei of all cells and incubated for at least 4 h or overnight and washed. The different cell types were counted using ImageJ cell counter; n =6–14 naive networks (3–7 cell extractions × 2 replicates each) and n =4 ARA-C treated cultures (two cell extractions × 2 replicates each) were evaluated. For activity imaging, cultures were incubated for 2–2.5 h at 37 °C with the organic calcium indicator Fluo-4 (2–3 μl ml −1 of a 1 μg μl −1 solution, Invitrogen). SLITE raw data consisted of planar images at different depths and time points. Images were grouped according to their axial position and cell segmentation for each plane was performed using CellProfiler (cells with centre position in adjacent planes were merged) or Imaris. Fluorescence signals were normalized according to , where F 0 is each cell’s average signal during the experiment’s first 30 s (after removing dark current), and F ( t ) is its temporal fluorescence signal. The identification of calcium transients was performed semi-automatically: a peak detection software (Peakdet Matlab function) performed initial analysis and a user manually added or cancelled detected peaks. Structural imaging of network development Cell cultures were transfected at DIV2 with lentiviral vectors encoding for Cerulean:SV2 (ref. 46 ) and PSD95:EGFP [32] . Time-lapse imaging were performed at 37 °C and controlled CO 2 conditions (protocol given in ref. 32 ) at DIV17–30 for 3–5 days using a custom-built Confocal Laser Scanning Microscope based on a Zeiss AxioObserver.Z1 using a 40 × 1.3 NA Fluar objective. Cultures were imaged every 30 or 60 min by averaging 4–6 images collected at each of 10 focal planes spaced 0.8 μm apart. How to cite this article: Dana, H. et al. Hybrid multiphoton volumetric functional imaging of large-scale bioengineered neuronal networks. Nat. Commun. 3:3997 doi: 10.1038/ncomms4997 (2014).